Mepenzolate bromide displays beneficial effects in a mouse model of chronic obstructive pulmonary disease The clinical treatment of chronic obstructive pulmonary disease (COPD) requires not only an improvement of airflow by bronchodilation but also the suppression of emphysema by controlling inflammation. Here we screen a compound library consisting of clinically used drugs for their ability to prevent elastase-induced airspace enlargement in mice. We show that intratracheal administration or inhalation of mepenzolate bromide, a muscarinic antagonist used to treat gastrointestinal disorders, decreases the severity of elastase-induced airspace enlargement and respiratory dysfunction. Although mepenzolate bromide shows bronchodilatory activity, most other muscarinic antagonists do not improve elastase-induced pulmonary disorders. Apart from suppressing elastase-induced pulmonary inflammatory responses and the production of superoxide anions, mepenzolate bromide reduces the level of cigarette smoke-induced airspace enlargement and respiratory dysfunction. Based on these results, we propose that mepenzolate bromide may be an effective therapeutic for the treatment of COPD due to its anti-inflammatory and bronchodilatory activities. Chronic obstructive pulmonary disease (COPD) is a serious health problem whose most important etiologic factor is cigarette smoke (CS) [1] . COPD is a disease that is defined by a progressive and partially reversible airflow limitation associated with abnormal inflammatory responses and permanent enlargement of the pulmonary airspace [1] , [2] , [3] . Thus, for the clinical treatment of COPD, it is important not only to improve the airflow limitation by bronchodilation, but also to suppress disease progression by controlling inflammatory processes. Bronchodilators (β 2 -agonists and muscarinic antagonists) are currently used for the treatment of COPD, providing an effective temporary improvement of airflow limitation [2] , [4] , [5] . On the other hand, steroids are used to suppress the inflammatory responses associated with COPD. However, steroids cannot significantly modulate disease progression and mortality [5] , [6] because the inflammation associated with COPD shows resistance to steroid treatment [7] . In addition to the fact that CS contains a high concentration of reactive oxygen species (ROS), activated leukocytes also produce large amounts of ROS, with one such example being the superoxide anions produced via the activation of nicotinamide adenine dinucleotide phosphate (NADPH) oxidase [8] . In contrast to this, the body contains a number of endogenous antioxidant proteins such as superoxide dismutase (SOD) and glutathione S- transferase (GST), with a decrease in these proteins reported to be involved in the pathogenesis of COPD [9] , [10] . The inflammatory responses associated with COPD are thought to be triggered by oxidative stress and mediated through the activation of nuclear factor-κB (NF-κB, a pro-inflammatory transcription factor) and inhibition of histone deacetylase 2 (HDAC2) [11] , [12] , [13] , [14] . Oxidative stress seems to activate NF-κB through the inhibition of HDAC activity and degradation of inhibitor of NF-κB (IκB)-α (refs 12 , 14 , 15 ). Pro-inflammatory gene expression is normally silenced by the condensation of DNA; however, the acetylation of core histones opens up the condensed chromatin and induces the expression of these genes (refs 11 , 12 , 16 ). HDACs suppress the expression of pro-inflammatory genes not only by maintaining chromatin condensation but also by directly modifying pro-inflammatory transcription factors (such as NF-κB) [12] . Moreover, HDACs, and particularly HDAC2, seem to have important roles in the inflammatory responses associated with COPD [11] , [17] , [18] . Furthermore, because corticosteroids use HDAC2 to suppress the activity of NF-κB [11] , [12] , [19] , the inhibitory effect of CS on HDAC2 may be responsible for the reduced sensitivity of COPD patients to steroid treatment [11] . Therefore, compounds that activate HDAC2 or inhibit ROS production and NF-κB may be effective for the treatment of inflammation associated with COPD. In the present study, we screen compounds that prevent elastase-induced airspace enlargement in mice from a library of existing medicines whose safety properties have already been well characterized in humans. We select mepenzolate bromide (mepenzolate), which is an orally administered muscarinic receptor antagonist used to treat gastrointestinal disorders [20] , [21] , [22] , and administer this compound to mice, which suppresses elastase-induced pulmonary inflammatory responses, airspace enlargement, alteration of lung mechanics and respiratory dysfunction. We also found that mepenzolate has bronchodilatory activity. These results suggest that mepenzolate achieves its anti-inflammatory effect via muscarinic receptor-independent inhibitory effects on NF-κB and NADPH oxidase, together with stimulatory effects on HDAC2, SOD and GST. We suggest that mepenzolate could provide an effective treatment option for COPD, not only as a consequence of its bronchodilatory activity but also due to its anti-inflammatory properties. Effect of mepenzolate on airspace enlargement From a group of 83 medicines already in clinical use ( Supplementary Table S1 ), we screened for compounds able to suppress porcine pancreatic elastase (PPE)-induced airspace enlargement. Each drug was administered intraperitoneally to mice, and after selecting eight candidate compounds based on the level of suppression of airspace enlargement ( Supplementary Table S1 ), these were administered intratracheally at various doses and their inhibitory effects on PPE-induced airspace enlargement evaluated. Following this process, mepenzolate was selected based on the level of suppression of airspace enlargement it provided at clinical dose or less. Histopathological analysis of pulmonary tissue using hematoxylin and eosin (H&E) staining revealed that PPE administration induced airspace enlargement (increase in the mean linear intercept (MLI)) and that the simultaneous daily intratracheal administration of mepenzolate suppressed this enlargement in a dose-dependent manner ( Fig. 1a,b ). 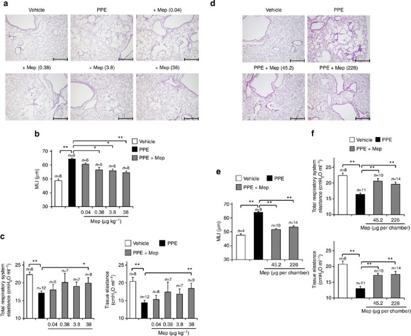Figure 1: Effect of mepenzolate on PPE-induced pulmonary disorders. Mice were treated with PPE (100 μg per mouse) once only on day 0 or with the vehicle only. The indicated doses (a–c, μg kg−1;d–f, μg per chamber) of mepenzolate (Mep) were administered intratracheally (a–c) or by inhalation (d–f) once daily for 14 days (from day 0 to day 13). Sections of pulmonary tissue were prepared on day 14 and subjected to histopathological examination (H&E staining) (scale bar, 500 μm) (a,d). Airspace size was estimated by determining the MLI as described in the Materials and Methods (b,e). Total respiratory system elastance and tissue elastance were determined on day 14 as described in the Methods (c,f). Values represent the mean±s.e.m.*P<0.05; **P<0.01(Tukey test). Experiments were replicated at least two times. Figure 1: Effect of mepenzolate on PPE-induced pulmonary disorders. Mice were treated with PPE (100 μg per mouse) once only on day 0 or with the vehicle only. The indicated doses ( a – c , μg kg −1 ; d – f , μg per chamber) of mepenzolate (Mep) were administered intratracheally ( a – c ) or by inhalation ( d – f ) once daily for 14 days (from day 0 to day 13). Sections of pulmonary tissue were prepared on day 14 and subjected to histopathological examination (H&E staining) (scale bar, 500 μm) ( a , d ). Airspace size was estimated by determining the MLI as described in the Materials and Methods ( b , e ). Total respiratory system elastance and tissue elastance were determined on day 14 as described in the Methods ( c , f ). Values represent the mean±s.e.m. *P<0.05; **P<0.01 (Tukey test). Experiments were replicated at least two times. Full size image The alteration of lung mechanics associated with pulmonary emphysema is characterized by a decrease in elastance. Total respiratory system elastance (elastance of the whole lung, including the bronchi, bronchioles and alveoli) and tissue elastance (elastance of alveoli) were decreased by the PPE treatment in a manner that could be restored in part by the simultaneous administration of mepenzolate, again in a dose-dependent manner ( Fig. 1c ). We next examined the effect of mepenzolate administered by the inhalation route on the PPE-induced airspace enlargement and alteration of lung mechanics. The results obtained ( Fig. 1d–f ) were similar to those observed with the intratracheal mode of administration ( Fig. 1a–c ). To determine the effect of mepenzolate on pre-developed pulmonary emphysema, the intratracheal administration of mepenzolate to mice was commenced 14 days after the administration of PPE, and airspace enlargement and lung mechanics were assessed on day 21. Compared with vehicle-treated animals, mepenzolate decreased the extent of PPE-induced airspace enlargement and alterations to lung mechanics ( Fig. 2a–c ), suggesting that mepenzolate could be an effective compound for the treatment of pre-developed pulmonary emphysema. 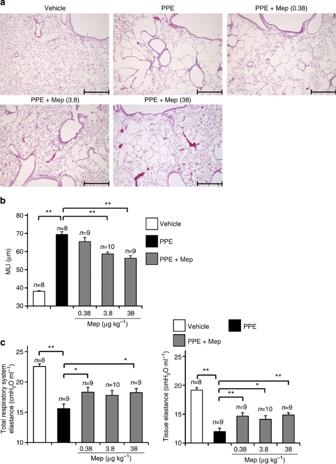Figure 2: Effect of mepenzolate on pre-developed pulmonary emphysema. Mice were treated with PPE (100 μg per mouse) once only on day 0 or with the vehicle only. The indicated doses (μg kg−1) of mepenzolate (Mep) were administered intratracheally once daily from day 14 to day 20. Sections of pulmonary tissue were prepared on day 21 and subjected to histopathological examination (H&E staining) (scale bar, 500 μm) (a). Airspace size was estimated by determining the MLI as described in the Materials and Methods (b). Total respiratory system elastance and tissue elastance were determined on day 21 as described in the Methods (c). Values represent the mean±s.e.m.*P<0.05; **P<0.01(Tukey test). Experiments were replicated at least two times. Figure 2: Effect of mepenzolate on pre-developed pulmonary emphysema. Mice were treated with PPE (100 μg per mouse) once only on day 0 or with the vehicle only. The indicated doses (μg kg −1 ) of mepenzolate (Mep) were administered intratracheally once daily from day 14 to day 20. Sections of pulmonary tissue were prepared on day 21 and subjected to histopathological examination (H&E staining) (scale bar, 500 μm) ( a ). Airspace size was estimated by determining the MLI as described in the Materials and Methods ( b ). Total respiratory system elastance and tissue elastance were determined on day 21 as described in the Methods ( c ). Values represent the mean±s.e.m. *P<0.05; **P<0.01 (Tukey test). Experiments were replicated at least two times. Full size image Effects of other muscarinic antagonists We next examined the effects of other muscarinic antagonists on PPE-induced airspace enlargement and alterations of lung mechanics. Even at the highest dose, none of muscarinic antagonists tested significantly suppressed the PPE-induced airspace enlargement or alterations in lung mechanics ( Fig. 3a–c ). 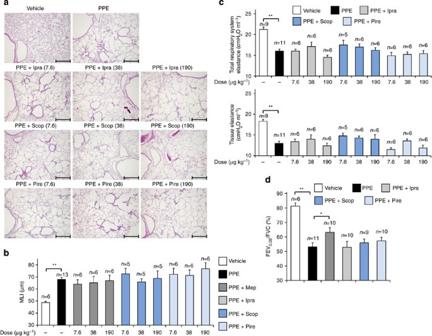Figure 3: Effect of different muscarinic antagonists on PPE-induced pulmonary disorders. Mice were treated with PPE (100 μg per mouse) once only on day 0 or with the vehicle only. The indicated doses (μg kg−1) (a–c) or 38 μg kg−1(d) of ipratropium (Ipra) (a–d), scopolamine (Scop) (a–d), pirenzepine (Pire) (a–d) or mepenzolate (Mep) (d) were administered intratracheally once daily for 14 days (from day 0 to day 13) (a–c) or for 11 days (from day 0 to day 10) (d). Sections of pulmonary tissue were prepared on day 14 and subjected to histopathological examination (H&E staining) (scale bar, 500 μm) (a). Airspace size was estimated by determining the MLI as described in the Materials and Methods (b). Total respiratory system elastance and tissue elastance were determined on day 14 as described in the Methods (c). The FEV0.05/FVC was determined on day 14 as described in the Materials and Methods (d). Values represent the mean±s.e.m.*P<0.05; **P<0.01(Tukey test). Experiments were replicated at least two times. Figure 3: Effect of different muscarinic antagonists on PPE-induced pulmonary disorders. Mice were treated with PPE (100 μg per mouse) once only on day 0 or with the vehicle only. The indicated doses (μg kg −1 ) ( a – c ) or 38 μg kg −1 ( d ) of ipratropium (Ipra) ( a – d ), scopolamine (Scop) ( a – d ), pirenzepine (Pire) ( a – d ) or mepenzolate (Mep) ( d ) were administered intratracheally once daily for 14 days (from day 0 to day 13) ( a – c ) or for 11 days (from day 0 to day 10) ( d ). Sections of pulmonary tissue were prepared on day 14 and subjected to histopathological examination (H&E staining) (scale bar, 500 μm) (a). Airspace size was estimated by determining the MLI as described in the Materials and Methods ( b ). Total respiratory system elastance and tissue elastance were determined on day 14 as described in the Methods ( c ). The FEV 0.05 /FVC was determined on day 14 as described in the Materials and Methods ( d ). Values represent the mean±s.e.m. *P<0.05; **P<0.01 (Tukey test). Experiments were replicated at least two times. Full size image The diagnosis of COPD is confirmed by a decrease in the ratio of forced expiratory volume in the first second (FEV 1 ) to forced vital capacity (FVC) [1] . We recently established a technique to monitor PPE-induced respiratory dysfunction in mice, and found that the FEV 0.05 /FVC ratio clearly decreased in PPE-treated mice compared with control mice [23] . Using this technique, we examined here the effects of mepenzolate and other muscarinic antagonists on the PPE-induced decrease in FEV 0.05 /FVC. To washout the bronchodilatory effect of the muscarinic antagonists, the administration of each drug was discontinued on day 10 and the assay performed on day 14. PPE treatment decreased the FEV 0.05 /FVC ratio, whereas the simultaneous administration of mepenzolate, but not the other muscarinic antagonists, restored the FEV 0.05 /FVC towards control values ( Fig. 3d ). The results in Fig. 3 show that ipratropium bromide (ipratropium), scopolamine N -butylbromide (scopolamine) and pirenzepine dihydrochloride (pirenzepine) were not effective in combatting PPE-induced airspace enlargement, nor did they improve lung mechanics or respiratory dysfunction. This finding suggests that mepenzolate achieves its ameliorative effect over PPE-induced pulmonary disorders via mechanisms that are independent of its effects on muscarinic receptors and bronchodilatory activity. To further test this idea, we examined the bronchodilatory activity induced by the muscarinic antagonists mentioned above. As shown in Fig. 4a , the dose-dependent increase in airway resistance (bronchoconstriction) induced by inhaled methacholine was completely suppressed by the intratracheal pre-administration of mepenzolate, thus attesting to the latter’s bronchodilatory activity. The dose-response profile of ipratropium for bronchodilation was similar to that of mepenzolate ( Fig. 4a ), although ipratropium had no effect against the PPE-induced pulmonary disorders ( Fig. 3 ). Neither scopolamine nor pirenzepine showed bronchodilatory activity, at least not at the highest dose employed here ( Supplementary Fig. S1 ). These results further support the notion that mepenzolate achieves its ameliorative effect against PPE-induced pulmonary disorders via muscarinic receptor- and bronchodilatory activity-independent mechanisms. In addition, the results in Fig. 4b show that, as for ipratropium, the bronchodilatory activity of mepenzolate was transient, diminishing 48 h after its administration. 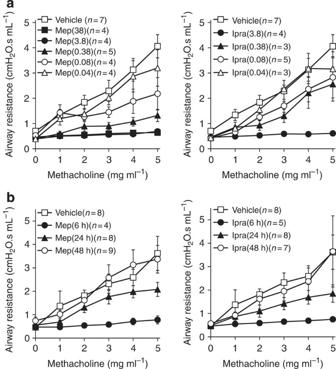Figure 4: Effect of mepenzolate on methacholine-induced airway constriction. Indicated doses (μg kg−1) (a) or 38 μg kg−1(b) of mepenzolate (Mep) or ipratropium (Ipra) were administered intratracheally. After 1 h (a) or indicated period (b), mice were exposed to nebulized methacholine five times and airway resistance was determined after each methacholine challenge as described in the Materials and Methods. Values are mean±s.e.m. Experiments were replicated at least two times. Figure 4: Effect of mepenzolate on methacholine-induced airway constriction. Indicated doses (μg kg −1 ) ( a ) or 38 μg kg −1 ( b ) of mepenzolate (Mep) or ipratropium (Ipra) were administered intratracheally. After 1 h ( a ) or indicated period ( b ), mice were exposed to nebulized methacholine five times and airway resistance was determined after each methacholine challenge as described in the Materials and Methods. Values are mean±s.e.m. Experiments were replicated at least two times. Full size image Muscarinic antagonists used to treat COPD are categorized as being long acting (such as tiotropium bromide (tiotropium) and glycopyrronium bromide (glycopyrronium)) or short acting (such as ipratropium), with the long-acting muscarinic antagonists now considered the standard bronchodilator treatment for COPD [24] . We subsequently examined the effect of intratracheal administration of tiotropium or glycopyrronium on PPE-induced pulmonary disorders. As shown in Supplementary Fig. S2a–c , glycopyrronium suppressed the PPE-induced airspace enlargement and alterations of lung mechanics. However, the extent of amelioration of airspace enlargement was not as apparent as that seen with mepenzolate ( Supplementary Fig. S2b ), and glycopyrronium did not significantly suppress the PPE-induced respiratory dysfunction ( Supplementary Fig. S2d ). On the other hand, tiotropium did not suppress the PPE-induced airspace enlargement, alterations of lung mechanics or respiratory dysfunction (except for a weak suppression of tissue elastance at the 30 μg kg −1 dose) ( Supplementary Fig. S2a–d ). Effect of mepenzolate on inflammatory responses We next monitored PPE-induced pulmonary inflammatory responses by determining the number of leucocytes in bronchoalveolar lavage fluid (BALF) 24 h after the administration of PPE. As shown in Fig. 5a , the total number of leucocytes and individual number of neutrophils were increased by the PPE treatment and this effect was suppressed by the simultaneous administration of mepenzolate. We also examined the levels of pro-inflammatory cytokines (tumour necrosis factor-α) and chemokines (macrophage inflammatory protein-2, monocyte chemoattractant protein-1 and keratinocyte-derived chemokine) in BALF. Levels of these pro-inflammatory cytokines and chemokines increased after the PPE treatment, and this increase was suppressed by the simultaneous treatment of animals with mepenzolate ( Fig. 5b ). These results suggest that mepenzolate could achieve its ameliorative effect by suppressing PPE-induced inflammatory responses. 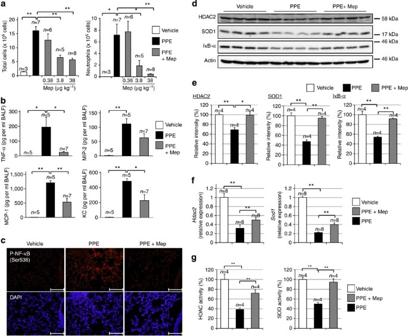Figure 5: Effect of mepenzolate on PPE-induced inflammatory responses. Indicated doses (μg kg−1) of mepenzolate (Mep) were administered intratracheally once only. Mice were treated with or without (vehicle) PPE (100 μg per mouse) 1 h after the mepenzolate administration. Twenty-four hours after the PPE administration, BALF (a,b), sections (c) or homogenates (d–g) were prepared from the lung. The total cell number and the number of neutrophils (a) or levels of cytokines and chemokines (b) were determined as described in the Materials and Methods. Immunohistochemical analysis with an antibody against the Ser536-phosphorylated form of NF-κB was performed as described in the Materials and Methods (scale bar, 100 μm) (c). Samples were analysed by immunoblotting with antibodies against HDAC2, SOD1, IκB-α or actin (d). The band intensity of each protein was determined and normalized with respect to actin (e). Total RNA was extracted and subjected to real-time RT-PCR using a specific primer set for each gene. Values were normalized to theGapdhgene and expressed relative to the control sample (f). The activity of HDAC or SOD was determined as described in the Materials and Methods (g). Values represent the mean±s.e.m.*P<0.05; **P<0.01(Tukey test). Experiments were replicated at least two times. Figure 5: Effect of mepenzolate on PPE-induced inflammatory responses. Indicated doses (μg kg −1 ) of mepenzolate (Mep) were administered intratracheally once only. Mice were treated with or without (vehicle) PPE (100 μg per mouse) 1 h after the mepenzolate administration. Twenty-four hours after the PPE administration, BALF ( a , b ), sections ( c ) or homogenates ( d – g ) were prepared from the lung. The total cell number and the number of neutrophils ( a ) or levels of cytokines and chemokines ( b ) were determined as described in the Materials and Methods. Immunohistochemical analysis with an antibody against the Ser536-phosphorylated form of NF-κB was performed as described in the Materials and Methods (scale bar, 100 μm) ( c ). Samples were analysed by immunoblotting with antibodies against HDAC2, SOD1, IκB-α or actin ( d ). The band intensity of each protein was determined and normalized with respect to actin ( e ). Total RNA was extracted and subjected to real-time RT-PCR using a specific primer set for each gene. Values were normalized to the Gapdh gene and expressed relative to the control sample ( f ). The activity of HDAC or SOD was determined as described in the Materials and Methods ( g ). Values represent the mean±s.e.m. *P<0.05; **P<0.01 (Tukey test). Experiments were replicated at least two times. Full size image We then focused on NF-κB and its regulator, HDAC2. The level of the Ser536-phosphorylated (active) form of NF-κB detected by immunohistochemical analysis increased in response to the PPE treatment, and could be suppressed by the simultaneous treatment of animals with mepenzolate ( Fig. 5c ). The level of IκB-α was decreased by the PPE treatment and remained stable when mepenzolate was concomitantly administered ( Fig. 5d,e ). As shown in Fig. 5f , Hdac2 mRNA expression was suppressed by the PPE treatment and could be partially restored by the simultaneous treatment of animals with mepenzolate. This alteration was also observed at the protein level ( Fig. 5d,e ). Furthermore, the enzymatic activity of HDAC was also decreased by the PPE treatment and could be partially restored by the simultaneous administration of mepenzolate ( Fig. 5g ). These results suggest that mepenzolate achieves its anti-inflammatory activity by increasing or decreasing the activity of HDAC2 or NF-κB, respectively. Effect of mepenzolate on superoxide anion production Electron spin resonance (ESR) analysis was employed to examine the effect of mepenzolate on the production of superoxide anions in mice. As shown in Fig. 6a,b , the peak amplitude corresponding to the superoxide anion level was higher in cells prepared from PPE-administered mice than in those from control mice. The peak amplitude in cells prepared from mice administered both PPE and mepenzolate was lower than that of mice administered PPE only ( Fig. 6a,b ), suggesting that mepenzolate suppresses the PPE-induced production of superoxide anions in the lung. The NADPH oxidase activity of cells in BALF was increased by the PPE treatment and could be partially suppressed by the simultaneous treatment of animals with mepenzolate ( Fig. 6c ). This suppression was observed at 4, 8 and 24 h but not 1 h after the administration of mepenzolate ( Fig. 6c ), suggesting that mepenzolate is a modulator of NADPH activation, but not an enzyme inhibitor of NADPH oxidase. On the other hand, the mRNA and protein expression of SOD1 and the enzymatic activity of SOD in the lung were decreased by the PPE treatment, with these effects also suppressed by the simultaneous administration of mepenzolate ( Fig. 5d–g ). These results suggest that mepenzolate suppresses the PPE-induced increase in superoxide anion production by modulating the activation of NADPH oxidase or activating SOD1. 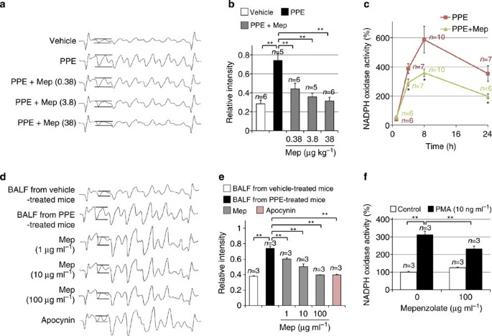Figure 6: Effect of mepenzolate on superoxide anion production. (a–c), indicated doses (μg kg−1) of mepenzolate (Mep) were administered intratracheally once only. Mice were treated with or without (vehicle) PPE (100 μg per mouse) 1 h after the mepenzolate administration. Cells in BALF were prepared 24 h (a,b) or 1, 4, 8, 24 h (c) after the PPE administration. Cells were incubated with a spin trap agent (DPhPMPO) for 10 min and subjected to radical adduct ESR spectrum analysis to determine the amount of superoxide anions present. The intensity of the ESR signal of the superoxide anion adduct (DPhPMPO-OOH adduct shown by the separation between the bars in the spectra shown in (a)) was determined (b). NADPH oxidase activities in cells were determined as described in the Materials and Methods and expressed relative to vehicle-treated controls (c). (d–f), mice were treated once only with or without (vehicle) PPE (100 μg per mouse) and cells in BALF were collected 24 h later. Cells were incubated with DPhPMPO in the presence of indicated concentrations of mepenzolate (μg ml−1) or 100 μM apocynin for 60 min. The level of superoxide anions was determined as described above (d,e). Cells were pre-incubated with or without mepenzolate (100 μg ml−1) for 3 h and further incubated with NADPH in the presence or absence of PMA (10 ng ml−1) for 20 min. NADPH oxidase activity was determined as described above (f). Values represent the mean±s.e.m.*P<0.05; **P<0.01(Tukey test). Experiments were replicated at least two times. Figure 6: Effect of mepenzolate on superoxide anion production. ( a – c ), indicated doses (μg kg −1 ) of mepenzolate (Mep) were administered intratracheally once only. Mice were treated with or without (vehicle) PPE (100 μg per mouse) 1 h after the mepenzolate administration. Cells in BALF were prepared 24 h ( a , b ) or 1, 4, 8, 24 h ( c ) after the PPE administration. Cells were incubated with a spin trap agent (DPhPMPO) for 10 min and subjected to radical adduct ESR spectrum analysis to determine the amount of superoxide anions present. The intensity of the ESR signal of the superoxide anion adduct (DPhPMPO-OOH adduct shown by the separation between the bars in the spectra shown in ( a )) was determined ( b ). NADPH oxidase activities in cells were determined as described in the Materials and Methods and expressed relative to vehicle-treated controls ( c ). ( d – f ), mice were treated once only with or without (vehicle) PPE (100 μg per mouse) and cells in BALF were collected 24 h later. Cells were incubated with DPhPMPO in the presence of indicated concentrations of mepenzolate (μg ml −1 ) or 100 μM apocynin for 60 min. The level of superoxide anions was determined as described above ( d , e ). Cells were pre-incubated with or without mepenzolate (100 μg ml −1 ) for 3 h and further incubated with NADPH in the presence or absence of PMA (10 ng ml −1 ) for 20 min. NADPH oxidase activity was determined as described above ( f ). Values represent the mean±s.e.m. *P<0.05; **P<0.01 (Tukey test). Experiments were replicated at least two times. Full size image We subsequently tested whether mepenzolate directly affects superoxide anion production in vitro . Cells prepared from the BALF of PPE-treated mice were incubated with a spin trap agent in the presence or absence of mepenzolate. As shown in Fig. 6d,e , mepenzolate decreased the level of superoxide anions in a dose-dependent manner, the extent of which was similar to that seen with apocynin (an inhibitor of NADPH oxidase). We found that the intratracheal administration of apocynin partially suppressed PPE-induced airspace enlargement and alterations of lung mechanics ( Supplementary Fig. S3 ). These findings suggest that most of the superoxide anions were produced by NADPH oxidase under these conditions and that mepenzolate could modulate NADPH oxidase activity and thus reduce the production of superoxide anions and PPE-induced pulmonary disorders. To understand the mechanism of the inhibitory effect of mepenzolate on NADPH oxidase activity, we examined the effect of mepenzolate on the PPE-dependent alteration of mRNA expression of genes related to NADPH oxidase (such as p91 phox (Nox2), p22 phox , p40 phox , p47 phox , p67 phox and Rac2 ). As shown in Supplementary Fig. S4a , PPE treatment upregulated the mRNA expression of these genes in a manner that could be suppressed by concomitant administration of mepenzolate. The mRNA expression of some of other Noxs ( Nox1, 4 ) and dual oxidases ( Duoxs ; Duox1, 2 ) was also affected by treatment with PPE and/or mepenzolate ( Supplementary Fig. S4b ). Furthermore, treatment of cells in BALF with phorbol 12-myristate 13-acetate (PMA) activated NADPH oxidase, whereas pretreatment of cells with mepenzolate decreased this activity in the presence of PMA treatment but not in its absence ( Fig. 6f ). This finding supports the notion that mepenzolate is a modulator of NADPH activation, but not an enzyme inhibitor of NADPH oxidase. Taken together, these results suggest that the modulatory effect of mepenzolate on NADPH oxidase activity can be explained in terms of its downmodulation of the expression of NADPH oxidase-related genes and the activation of this enzyme. To further understand the mechanism governing the mepenzolate-dependent decrease in inflammatory responses and oxidative stress, we performed DNA microarray analysis of lung tissue from mepenzolate-treated (or control) mice. Among the genes whose expression was altered by the mepenzolate administration ( Table 1 ), we focused on genes encoding GSTs that were included in a ‘glutathione metabolism’ gene set ( Supplementary Fig. S5a,b ) and are known to reduce oxidative stress by decreasing lipid peroxide levels [9] . As shown in Fig. 7a,b , the mRNA expression of Gst genes and GST activity in the lung were increased by the mepenzolate administration. The mepenzolate administration also restored GST activity, which was decreased by the PPE treatment ( Fig. 7c ). It was reported that GST and its regulatory transcription factor, NF-E2-related factor 2 (Nrf2), in macrophages have an important role in the pathogenesis of COPD [25] , [26] . Therefore, we performed the Gene Set Enrichment Analysis using the custom gene set and confirmed that the downstream genes of Nrf2 (NFE2L2 target genes) were upregulated by the mepenzolate administration ( Supplementary Fig. S5c,d ). Furthermore, we found that treatment of RAW264 cells (a macrophage cell line) with mepenzolate upregulated the mRNA expression Gst genes and GST activity ( Fig. 7d,e ). Mepenzolate also activated Nrf2 and the expression of other Nrf2-regulated genes (heme oxygenase 1 ( Ho1), NAD(P)H dehydrogenase, quinone1 (Nqo1) and Sod1 ) in RAW264 cells ( Fig. 7f,g ). These results suggest that the stimulatory effect of mepenzolate on Nrf2 activity and the resulting expression of Gst genes also involve the mepenzolate-dependent decrease in inflammatory responses and oxidative stress. Table 1 List of gene sets that were differently expressed at 25 h after administration of mepenzolate. 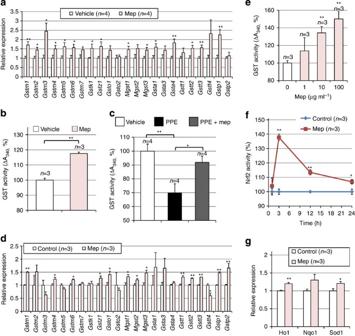Figure 7: Effect of mepenzolate onGstgene expression and GST activity. (a–c), mepenzolate (Mep) (38 μg kg−1) or vehicle (PBS) was administered intratracheally once only. Mice were treated with or without PPE (100 μg per mouse) 1 h after the mepenzolate administration (c). Twenty-five hours after the mepenzolate administration, lung homogenates was prepared. Total RNA was extracted and subjected to real-time RT-PCR using a specific primer set for each gene. Values were normalized to theHprtgene and expressed relative to the control sample (a). The GST activity was determined as described in the Materials and Methods and expressed relative to the control sample (b,c). (d–g), RAW264 cells were incubated for 24 h (d,e,g) or indicated period (f) with or without (control) 100 μg ml−1(d,f,g) or indicated doses (e) of mepenzolate (Mep). The mRNA expression of each gene was monitored as described above (d,g). Activities of GST and Nrf2 were determined as described in the Materials and Methods and expressed relative to the control sample (e,f). Values represent the mean±s.e.m.*P<0.05; **P<0.01(Student’st-test (a,b,d–g), Tukey test (c)). Experiments were replicated at least two times. Full size table Figure 7: Effect of mepenzolate on Gst gene expression and GST activity. ( a – c ), mepenzolate (Mep) (38 μg kg −1 ) or vehicle (PBS) was administered intratracheally once only. Mice were treated with or without PPE (100 μg per mouse) 1 h after the mepenzolate administration ( c ). Twenty-five hours after the mepenzolate administration, lung homogenates was prepared. Total RNA was extracted and subjected to real-time RT-PCR using a specific primer set for each gene. Values were normalized to the Hprt gene and expressed relative to the control sample ( a ). The GST activity was determined as described in the Materials and Methods and expressed relative to the control sample ( b , c ). ( d – g ), RAW264 cells were incubated for 24 h ( d , e , g ) or indicated period ( f ) with or without (control) 100 μg ml −1 ( d , f , g ) or indicated doses ( e ) of mepenzolate (Mep). The mRNA expression of each gene was monitored as described above ( d , g ). Activities of GST and Nrf2 were determined as described in the Materials and Methods and expressed relative to the control sample ( e , f ). Values represent the mean±s.e.m. *P<0.05; **P<0.01 (Student’s t -test ( a , b , d – g ), Tukey test ( c )). Experiments were replicated at least two times. Full size image Effect of mepenzolate on CS-induced pulmonary disorders Finally, we examined the effect of the intratracheal administration of mepenzolate on CS-induced pulmonary disorders. As shown in Fig. 8a–c , pulmonary inflammatory responses and airspace enlargement were induced following exposure of mice to CS, with the simultaneous intratracheal administration of mepenzolate clearly suppressing the severity of these CS-induced pulmonary disorders. We also found that the exposure of mice to CS decreased total respiratory system elastance and tissue elastance and that these parameters could be clearly improved by the simultaneous administration of mepenzolate ( Fig. 8d ). Administration of mepenzolate also suppressed CS-induced increases in oxidative stress (the pulmonary level of 8-hydroxy-2′-deoxyguanosine (8-OHdG)) ( Fig. 8e ). Mepenzolate increased GST activity in either the presence or absence of CS treatment in vivo ( Fig. 8f ) . In vitro , GST activity was increased by the treatment of cells with mepenzolate, even in the presence of CS extract (CSE), which itself activated GST ( Fig. 8g ). On the other hand, we found that mepenzolate suppressed the CS-induced mRNA expression of Mip-2 and Kc and activation of NADPH oxidase ( Supplementary Fig. S6a,b ). Mepenzolate also restored the HDAC and SOD activities that were decreased by exposure to CS ( Supplementary Fig. S6c ). These results suggest that mepenzolate protects against CS-induced pulmonary disorders via a mechanism similar to that in which it exerts its action against PPE-induced pulmonary disorders. 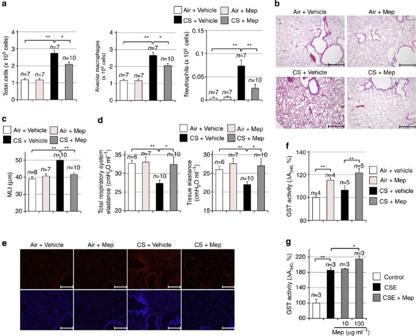Figure 8: Effect of mepenzolate on CS-induced pulmonary disorders. (a–f), mice were exposed to CS (three times per day) and intratracheally administered mepenzolate (Mep; 38 μg kg−1, once daily) for 3 days (a,f) or for 6 months (5 days per week (from Monday to Friday)) (b–e) as described in the Materials and Methods. Only CS exposure was performed in the last week (b–e). The total cell number and the number of neutrophils or macrophages were determined as described in the Materials and Methods (a). Sections of pulmonary tissue were subjected to histopathological examination (H&E staining) (scale bar, 500 μm) (b). Airspace size was estimated by determining the MLI as described in the Materials and Methods (c). Total respiratory system elastance and tissue elastance were determined as described in the Methods (d). Immunohistochemical analysis with an antibody against 8-OHdG was performed as described in the Materials and Methods (scale bar, 200 μm) (e). The GST activity was determined as described in the Materials and Methods (f). (g) RAW264 cells were pre-incubated for 24 h with indicated concentrations of mepenzolate (Mep) and further incubated with CSE (15%) for 24 h. GST activity was determined as described above. Values represent the mean±s.e.m.*P<0.05; **P<0.01(Tukey test). Experiments were replicated at least two times (except forb–e). Figure 8: Effect of mepenzolate on CS-induced pulmonary disorders. ( a – f ), mice were exposed to CS (three times per day) and intratracheally administered mepenzolate (Mep; 38 μg kg −1 , once daily) for 3 days ( a , f ) or for 6 months (5 days per week (from Monday to Friday)) ( b – e ) as described in the Materials and Methods. Only CS exposure was performed in the last week ( b – e ). The total cell number and the number of neutrophils or macrophages were determined as described in the Materials and Methods ( a ). Sections of pulmonary tissue were subjected to histopathological examination (H&E staining) (scale bar, 500 μm) ( b ). Airspace size was estimated by determining the MLI as described in the Materials and Methods ( c ). Total respiratory system elastance and tissue elastance were determined as described in the Methods ( d ). Immunohistochemical analysis with an antibody against 8-OHdG was performed as described in the Materials and Methods (scale bar, 200 μm) ( e ). The GST activity was determined as described in the Materials and Methods ( f ). ( g ) RAW264 cells were pre-incubated for 24 h with indicated concentrations of mepenzolate (Mep) and further incubated with CSE (15%) for 24 h. GST activity was determined as described above. Values represent the mean±s.e.m. *P<0.05; **P<0.01 (Tukey test). Experiments were replicated at least two times (except for b – e ). Full size image The number of drugs reaching the marketplace each year is decreasing, mainly because of the unexpected adverse effects of potential drugs being revealed at advanced stages of clinical trials. To circumvent this, we have proposed a new strategy for drug discovery and development, which focuses on the use of medicines that have already been approved for use by humans (drug repositioning) [27] . In this strategy, compounds with clinically beneficial pharmacological activity are screened from a library of medicines already in clinical use to be developed for new indications. The advantage of this strategy is that there is a decreased risk for unexpected adverse effects in humans because the safety aspects of these drugs have already been well characterized in humans [27] . In the present study, we applied this strategy to screen for drugs to combat COPD. The drug mepenzolate was identified using this approach, and we found that its intratracheal administration suppresses PPE-induced airspace enlargement and alteration of lung mechanics, suggesting that mepenzolate could provide an effective treatment for COPD. To highlight the potential clinical relevance of our findings, we performed several key experiments. First, we demonstrated that inhalation of mepenzolate was also effective against PPE-induced airspace enlargement and alteration of lung mechanics. This route of administration is noteworthy because of its potential to have less impact on the quality of life of COPD patients given that the drug can be administered on a daily basis at home. Second, we showed that mepenzolate has a therapeutic effect even when the drug was administered after the development of emphysema. We also showed that mepenzolate suppresses the PPE-induced decrease in FEV 0.05 /FVC and finally, we demonstrated that mepenzolate exerts an ameliorative effect against CS-induced pulmonary disorders. Among the five types of muscarinic receptors (M 1–5 R), M 3 R expressed in bronchial smooth muscle can be blocked by muscarinic antagonists, resulting in bronchodilation [28] . Thus, it is reasonable to speculate that mepenzolate, a subtype-non-specific muscarinic receptor antagonist, has bronchodilatory activity as confirmed here. Other subtype-non-specific muscarinic receptor antagonists such as ipratropium and tiotropium examined here did not exert ameliorative effects against PPE-induced pulmonary disorders. Furthermore, scopolamine (a subtype-non-specific muscarinic receptor antagonist) and pirenzepine (an M 1 R-specific antagonist) also had no discernible effects against PPE-induced pulmonary disorders, even though, as for mepenzolate, these drugs are orally administered drugs used to treat gastrointestinal disorders and their clinical doses (100 mg per day per adult) are similar to that of mepenzolate (45 mg per day per adult). We also found that the M 2 R-specific antagonist gallamine triethiodide and the M 3 R-specific antagonist 1,1-dimethyl-4-diphenylacetoxypiperidinium iodide did not affect the PPE-induced increase in number of total leukocytes or neutrophils in BALF ( Supplementary Fig. S7 ). These results suggest that mepenzolate achieves its ameliorative effect against PPE-induced pulmonary disorders via mechanisms that are independent of its muscarinic receptor and bronchodilatory activities. On the other hand, glycopyrronium suppressed PPE-induced airspace enlargement and alterations of lung mechanics. The chemical structure of glycopyrronium is similar to that of mepenzolate ( Supplementary Fig. S8 ), suggesting that this common structure may underlie their anti-inflammatory activities. Mepenzolate suppressed both PPE- and CS-induced inflammatory responses. We found that the pulmonary level of the active forms of NF-κB or IκB-α increased or decreased, respectively, in response to the treatment of mice with PPE, and that the simultaneous treatment of animals with mepenzolate partially suppressed these alterations. We also found that HDAC2 and HDAC activities were decreased by the PPE treatment of mice and that simultaneous treatment with mepenzolate partially suppressed these decreases. This finding suggests that NF-κB and HDAC2 have important roles in the inhibitory effect of mepenzolate on inflammatory responses. We also observed that treatment of mice with mepenzolate suppressed the PPE- induced increases in oxidative stress, NADPH oxidase activity and expression of NADPH oxidase-related genes. The incubation of cultured cells retrieved from BALF exhibited decreased superoxide anion production and PMA-induced activation of NADPH oxidase when the incubation was carried out in the presence of mepenzolate. However, mepenzolate did not affect the background level of NADPH oxidase activity. These results suggest that mepenzolate suppresses the PPE-induced production of superoxide anions via the modulation of NADPH oxidase activation and expression of NADPH oxidase-related genes. It was reported that polymorphisms in genes encoding GSTs affect the pathogenesis of COPD, [29] and we here found that mepenzolate increased the expression of Gst genes and GST activity in the lung. We also found that treatment of RAW264 cells with mepenzolate increased the expression of Gst genes and GST and Nrf2 activities. These results suggest that the mepenzolate-dependent decrease in the pulmonary level of oxidative stress in vivo also involves its stimulatory effect on Nrf2 and the resulting expression of Gst genes. It should be noted that both the modulatory effect of mepenzolate on NADPH oxidase activation and its stimulatory effect on the expression of Gst genes and GST activity seems not to be a secondary effect of alternative mechanisms, because these effects can be reproduced in vitro . Furthermore, the expression of SOD1 in the lung, which is regulated by Nrf2 (ref. 26 ), was decreased by the PPE treatment, and subsequently restored by the concomitant treatment of animals with mepenzolate. This action of mepenzolate may also be involved in the observed decreased oxidative stress in vivo . Oxidative stress activates NF-κB via both the inhibition of HDAC2 and the stimulation of IκB-α degradation, with these mechanisms suggested to be important for inflammatory responses associated with COPD [12] , [14] . Therefore, we conclude that mepenzolate suppresses inflammatory responses in animal models of COPD due to its inhibitory effect on ROS production, its stimulatory effect on the expression of antioxidant proteins and the resulting inhibition of NF-κB, which is caused by the activation of HDAC2 and the inhibition of IκB-α degradation. As described above, a combination of anti-inflammatory drugs (such as steroids) and bronchodilators is the standard treatment regime for COPD [30] , [31] . We have shown that mepenzolate has both anti-inflammatory and bronchodilatory activities, suggesting that this drug could be effective for the treatment of COPD without the concomitant use of other drugs. However, the results of this study suggest that mepenzolate belongs to the short-acting muscarinic antagonists, which are used as supplemental drugs for the temporary improvement of airflow limitation [24] . On the other hand, we recently reported that steroids do not provide protective or therapeutic benefits against PPE-induced pulmonary emphysema, alterations in lung mechanics or respiratory dysfunction [23] , whereas here we have shown that mepenzolate is effective against these disorders under the same experimental conditions. Based on these observations, we consider that a combination treatment regime involving the administration of long-acting muscarinic antagonists or β 2 -agonists along with inhaled mepenzolate may prove to be therapeutically beneficial for COPD patients. Chemicals and animals Mepenzolate, PPE, PMA, glycopyrronium, ipratropium, scopolamine, N, N′-dimethyl-9, 9′-biacridinium dinitrate (lucigenin), NADPH and acetyl-β-methylcholine bromide (methacholine) were obtained from Sigma (St Louis, MO). Antibodies against HDAC2, IκB-α, the Ser536-phosphorylated form of NF-κB and actin, along with apocynin were from Santa Cruz Biotechnology (Santa Cruz, CA). GeneChip Mouse Gene 1.0 ST Array was from Affymetrix (Santa Clara, CA). Alexa Fluor 594 goat anti-rabbit (or anti-mouse) immunoglobulin G was purchased from Invitrogen (Carlsbad, CA). Antibody against SOD1, gallamine triethiodide and 1,1-dimethyl-4-diphenylacetoxypiperidinium iodide and the HDAC assay kit were from Enzo Life Sciences (Farmingdale, NY). An antibody against 8-OHdG was from Nikken SEIL (Shizuoka, Japan). The GST assay kit was from PromoCell GmbH (Heidelberg, Germany). TransAM Nrf2 kit was from Active Motif (Carlsbad, CA). The SOD assay kit and the nuclear extraction hypotonic buffer were from Cayman Chemical (Ann Arbor, MI). Mounting medium for immunohistochemical analysis (VECTASHIELD) was from Vector Laboratories (Burlingame, CA). Novo-Heparin for injection was from Mochida Pharmaceutical (Tokyo, Japan). Chloral hydrate was from Nacalai Tesque (Kyoto, Japan). Diff-Quik was from the Sysmex Corporation (Kobe, Japan). ELISA kits for tumour necrosis factor-α, macrophage inflammatory protein-2, monocyte chemoattractant protein-1 and keratinocyte-derived chemokine were from R&D Systems (Minneapolis, MN). The RNeasy kit was obtained from Qiagen (Valencia, CA), the PrimeScript 1st strand cDNA Synthesis Kit was from TAKARA Bio (Ohtsu, Japan), and the SsoFast EvaGreen Supermix was from Bio-Rad (Hercules, CA). Pirenzepine dihydrochloride (pirenzepine) and formalin neutral buffer solution were from WAKO Pure Chemicals (Tokyo, Japan). Mayer’s hematoxylin, 1% eosin alcohol solution and malinol were from MUTO Pure Chemicals (Tokyo, Japan). DAPI, diethylenetriamine- N, N, N′, N′′, N′′ -pentaacetic acid and DPhPMPO were from Dojindo (Kumamoto, Japan). RAW264 cells (a macrophage cell line) were from RIKEN BioResource Center (Tsukuba, Japan). ICR mice (4–6 weeks old, male) and DBA/2 mice (5 weeks old, female) were purchased from Charles River (Yokohama, Japan) and used in all experiments in this paper. The experiments and procedures described here were carried out in accordance with the Guide for the Care and Use of Laboratory Animals as adopted and promulgated by the National Institutes of Health, and were approved by the Animal Care Committee of Keio University and Kumamoto University. Preparation of BALF and CSE and cell culture BALF was collected by cannulating the trachea and lavaging the lung with 1 ml of sterile PBS containing 50 units ml −1 heparin (two times). About 1.8 ml of BALF was routinely recovered from each animal. The total cell number was counted using a hemocytometer. Cells were stained with Diff-Quik reagents after centrifugation with Cytospin4 (Thermo Electron Corporation, Waltham, MA), and the ratio of neutrophils to total cell number was determined. Cells from BALF or RAW264 cells were cultured in Eagle’s minimal essential medium supplemented with 10% FBS or Eagle’s minimal essential medium supplemented with 10% FBS and 0.1 mM non-essential amino acid (Lonza, Allendale, NJ), respectively, in a humidified atmosphere of 95% air with 5% CO 2 at 37 °C. One cigarette (Peace; Japan Tobacco, Tokyo, Japan) was puffed 15 times over a 5 min period to obtain the smoke, which was bubbled into 5 ml of the culture medium using a 50-ml plastic syringe. The resulting suspension was defined 100% CSE [25] . Analyses of cytokines and chemokines and enzyme activities Cytokine and chemokine levels were measured by ELISA according to the manufacturer’s protocol. The activities of HDAC, SOD, GST and Nrf2 were measured by employing each assay kit according to the manufacturer’s protocol. For the measurement of Nrf2 activity, nuclear extract was prepared as described in the manufacturer’s protocol. Measurement of level of superoxide anions The level of superoxide anions was determined by ESR spin trapping with DPhPMPO [32] , [33] . Cells collected from BALF were incubated with 0.9% NaCl containing 500 μM diethylenetriamine- N, N, N′, N′′, N′′ -pentaacetic acid and 10 mM DPhPMPO for 10 min at 37 °C. ESR spectra were recorded at room temperature on a JES-TE200 ESR spectrometer (JEOL, Tokyo, Japan) under the following conditions: modulation frequency, 100 kHz; microwave frequency, 9.43 GHz; microwave power, 40 mW; scanning field, 330.2–340.2 mT; sweep time, 2 min; field modulation width, 0.25 mT; receiver gain, 400; and time count, 0.3 s. Every buffer and solution used in the reaction mixture used for ESR measurement was treated with Chelex 100 resin (Bio-Rad, Hercules, CA) before use to remove metal cations. The ESR spectrum was consistent with a previously reported DPhPMPO-OOH spectrum (a hyperfine coupling constant of a N =1.24 mT, =1.16 mT, a P =3.95 mT) [34] . Measurement of NADPH oxidase activity Cells in BALF were prepared as described above. NADPH oxidase activity in the cells was measured by using lucigenin as a substrate (chemiluminescence) [35] . Samples were incubated with 0.1 mM NADPH in 50 mM phosphate buffer containing 1 mM EGTA, 150 mM sucrose and 0.5 mM lucigenin, and lucigenin chemiluminescence was recorded for 15 min in a microplate reader (MicroLumat Plus LB96V, Berthold Technologies, Bad Wildbad, Germany or Infinite M1000, TECAN Group, Mannedorf, Switzerland). Histological and immunohistochemical analyses Lung tissue samples were fixed in 10% formalin neutral buffer solution for 24 h at a pressure of 25 cmH 2 O, and then embedded in paraffin before being cut into 4 μm-thick sections. For histological examination, sections were stained first with Mayer’s hematoxylin and then with 1% eosin alcohol solution (H&E staining). Samples were mounted with malinol and inspected with the aid of an Olympus BX51 microscope (Tokyo, Japan). To determine the MLI (an indicator of airspace enlargement), 20 lines (500 μm) were drawn randomly on the image of section stained with H&E and the intersection points with the alveolar walls were counted to determine the MLI. The morphometric analysis at the light microscopic level was conducted by an investigator blinded to the study protocol. For immunohistochemical analysis, sections were treated with 20 μg ml −1 protease K for antigen activation. Sections were blocked with 2.5% goat serum for 10 min, incubated for 12 h with an antibody against the Ser536-phosphorylated form of NF-κB (1:100 dilution) or 8-OHdG (1:100 dilution) in the presence of 2.5% bovine serum albumin, and then incubated for 2 h with Alexa Fluor 594 goat anti-rabbit (or anti-mouse) immunoglobulin G (1:500 dilution) and DAPI (5 μg ml −1 ). Samples were mounted with VECTASHIELD and inspected with the aid of a fluorescence microscope (Olympus BX51). Immunoblotting analysis Lung homogenates were prepared by homogenization in the buffer (50 mM Tris-HCl pH7.6, 150 mM NaCl, 1% NP-40, 1% sodium deoxycholate and 0.1% SDS) and the protein concentration of the samples was determined by the Bradford reagent [36] . Samples were applied to polyacrylamide SDS gels, subjected to electrophoresis and the resultant proteins immunoblotted with their respective antibodies. Full gel scans were shown in Supplementary Fig. S9 . Real-time RT–PCR analysis Total RNA was extracted from lung tissues using an RNeasy kit according to the manufacturer’s protocol. Samples (2.5 μg RNA) were reverse transcribed using a first-strand cDNA synthesis kit. Synthesized cDNA was used in real-time RT–PCR (Chromo 4 instrument (Bio-Rad, Hercules, CA) experiments using SsoFast EvaGreen Supermix, and analysed with Opticon Monitor Software. Specificity was confirmed by electrophoretic analysis of the reaction products and by inclusion of template- or reverse transcriptase-free controls. To normalize the amount of total RNA present in each reaction, glyceraldehyde-3-phosphate dehydrogenase or hypoxanthine guanine phosphoribosyltransferase cDNA was used as an internal standard. Primers were designed using the Primer3 or Primer-BLAST website. The primers sequence was shown in Supplementary Table S2 . Treatment of mice with PPE and CS ICR mice maintained under anaesthesia with chloral hydrate (500 mg kg −1 ) were given one intratracheal injection of PPE (100 μg per mouse or 15 U kg −1 ) in PBS via micropipette. DBA/2 or ICR mice were exposed to CS by placing 10–20 mice in a chamber (volume, 45 l) connected to a CS-producing apparatus. Commercial non-filtered cigarettes (Peace; Japan Tobacco, Tokyo, Japan) that yielded 28 mg tar and 2.3 mg nicotine on a standard smoking regimen were used. Mice were exposed to the smoke of 1 cigarette for 35 min, 3 times per day, 5 days per week (from Monday to Friday) for 6 months, or to the smoke of 2 cigarettes for 25 min, 3 times per day for 3 days. The apparatus was configured such that each cigarette was puffed 15 times over a 5-min period. For the administration of mepenzolate by inhalation, 5–8 mice were placed in a chamber (volume, 45 l) and an ultrasonic nebulizer (NE-U07, Omron, Tokyo, Japan) connected to the chamber was used to nebulize over a 30-min period the entire volume of a solution containing mepenzolate dissolved in 10 ml PBS. For control mice, PBS alone was nebulized. Mice were kept in the chamber for a further 10 min after completion of the nebulization. For the intratracheal administration of candidate drugs, mice were maintained under anaesthesia with chloral hydrate (500 mg kg −1 ) and each drug in PBS was administered via micropipette. For control mice, PBS alone was administered by the same procedure. Unless otherwise noted, the first administration of each drug was performed 1 h prior to the PPE administration or 2 h before the CS treatment. Analyses of lung mechanics and respiratory functions Measurement of lung mechanics and airway resistance was performed with a computer-controlled small-animal ventilator (FlexiVent, SCIREQ, Montreal, Canada) [32] , [33] . Mice were anesthetized with chloral hydrate (500 mg kg −1 ), a tracheotomy was performed, and an 8-mm section of metallic tube was inserted into the trachea. Mice were mechanically ventilated at a rate of 150 breaths per min, using a tidal volume of 8.7 ml kg −1 and a positive end-expiratory pressure of 2–3 cmH 2 O. Total respiratory system elastance and tissue elastance were measured by the snap shot and forced oscillation techniques, respectively. All data were analysed using FlexiVent software (version 5.3; SCIREQ, Montreal, Canada). For measurement of the methacholine-induced increase in airway resistance, mice were exposed to nebulized methacholine (1 mg ml −1 ) five times for 20 s with a 40-s interval between each and airway resistance was measured after each methacholine challenge by the snap shot technique. All data were analysed using the FlexiVent software. Determination of the FEV0.05/FVC ratio was performed with the same computer-controlled small-animal ventilator connected to a negative pressure reservoir (SCIREQ, Montreal, Canada) [32] , [33] . Mice were tracheotomized and ventilated as described above. The lungs were inflated to a pressure of 30 cm H 2 O over 1 s and held at this pressure. After 0.2 s, the pinch valve (connected to ventilator) was closed and after 0.3 s, the shutter valve (connected to negative pressure reservoir) was opened for exposure of the lung to the negative pressure. The negative pressure was held for 1.5 s to ensure complete expiration. FEV0.05/FVC was determined using the FlexiVent software. Gene expression analysis using DNA microarray Using 100 ng of total RNA extracted from lung tissues, hybridization and signal detection of GeneChip Mouse Gene 1.0 ST Arrays (Affymetrix, Santa Clara, CA) were performed following the manufacturer's instructions. Gene expression analysis was performed in duplicate for each experimental condition. The raw data were normalized by the robust multi-array average method [37] using the ‘affy’ package from BioConductor ( http://www.bioconductor.org/ ) and R statistical software version 2.12.1 ( http://www.r-project.org/ ). For functional analysis, we used Gene Set Enrichment Analysis version 2.0.13 with MSigDB gene sets version 4.0 (ref. 38 ). A gene set category c2.cp.kegg based on the KEGG pathway database was used, and a custom gene set (SINGH_NFE2L2_TARGETS from the category c2.cgp) was used for the analysis of Nrf2-related gene sets. We used ‘Diff_of_Classes’ (the difference of class means to calculate fold change) as a metric for ranking genes. All other parameters were set to the default values, except for ‘set_min’ (the minimum size of gene set) to 10 for the Nrf2-related gene sets. Gene sets satisfying P <0.05 and FDR<0.25 were considered significant. Statistical analysis All values are expressed as the mean±s.e.m. Two-way analysis of variance followed by the Tukey test or the Student’s t -test for unpaired results was used to evaluate differences between three or more groups or between two groups, respectively. Differences were considered to be significant for values of P <0.05. How to cite this article: Tanaka, K.-I. et al. Mepenzolate bromide displays beneficial effects in a mouse model of chronic obstructive pulmonary disease. Nat. Commun. 4:2686 doi: 10.1038/ncomms3686 (2013).